Logic gates based on ion transistors Precise control over processing, transport and delivery of ionic and molecular signals is of great importance in numerous fields of life sciences. Integrated circuits based on ion transistors would be one approach to route and dispense complex chemical signal patterns to achieve such control. To date several types of ion transistors have been reported; however, only individual devices have so far been presented and most of them are not functional at physiological salt concentrations. Here we report integrated chemical logic gates based on ion bipolar junction transistors. Inverters and NAND gates of both npn type and complementary type are demonstrated. We find that complementary ion gates have higher gain and lower power consumption, as compared with the single transistor-type gates, which imitates the advantages of complementary logics found in conventional electronics. Ion inverters and NAND gates lay the groundwork for further development of solid-state chemical delivery circuits. In ion transistors [1] , [2] , [3] , [4] , the charge carriers are represented by ions and charged molecules. As the mobility of these species is typically much lower than the mobility of the electrons and holes found in conventional semiconductors, ion transistors and circuits will never compete with traditional transistors in terms of speed. However, the species transported in ion transistors carry specific chemical information and functionality in themselves and can therefore selectively regulate various functions and processes. Thus, despite the limited speed, ion transistor circuits can be useful in delivering, regulating and establishing signalling patterns of ions and biomolecules. Applications and processes in which chemical circuits may be applicable include drug delivery [5] (timescale of interest ranging from minutes to days), neuromudulation [6] (seconds to hours), controlled polymerization [7] (minutes to hours), intracellular calcium oscillations [8] (microseconds to days) and plant development [9] (minutes to days). Ion transistors can be divided into two subgroups based on their principle of operation: field-effect transistors and bipolar junction transistors (BJTs) [10] . Nanofluidic transistors [1] are the major type of field effect ion transistors currently investigated, although other promising devices such as polysaccharide field-effect transistors [3] also are under development. In nanofluidic transistors, the conductivity within the ion transistor is modulated by field-induced surface charges along a narrow channel configuration. Unfortunately, the performance of these devices deteriorates with increasing salt concentration due to screening of the surface charges [11] (Debye screening length is ~1 nm at 100 mM salt concentration). Few publications have been reporting ion transistors based on the BJT principle. Nanofluidic bipolar transistors have been proposed [12] and fixed pnp -junctions was implemented in a polymer pore [13] ; however, both of these devices still operates in the field-effect mode compared with BJTs in which the conduction occurs throughout the bulk of the conductor. To overcome the limitations of surface charge modulation, we have previously developed another type of ion transistor, the ion bipolar junction transistor [4] , [14] (IBJT), which is based on thin layers of ion selective membranes [15] and conductive polymers [16] , [17] . IBJTs shows overall good transistor characteristics, in terms of, for instance, a high ion current on–off and gain, and have successfully been utilized to modulate the delivery of neurotransmitter to regulate signalling of neuronal cells [4] . To further develop applications based on IBJTs, individual transistors have to be integrated into circuits. A first natural step is to implement some of the basic logic functions, from which arbitrary logical expressions can be constructed. Previously, the AND gate has been implemented with ion diodes [18] , [19] ; however, there are several limitations associated with diode logics, including lack of gain and inability to achieve inversion, that is, NAND and NOT gates. Logics based on transistors do not posses these limitations, but till now, only theoretical predictions of ion transistor logics have been presented [20] . The field of electronics has established several ways of implementing logic gates, and the same schemes [21] can be utilized within the field of chemical circuits. In this work, we demonstrate the realization of the NOT and NAND gates with IBJTs. NAND gates are particularly important because they alone are sufficient to implement arbitrary logical expressions. Both gates are realized in a single transistor type ( npn -type) configuration as well as in a complementary ( npn - and pnp -type) fashion. Ion bipolar junction transistors IBJTs are built up from patterned films that are either cation or anion selective, corresponding to the p - and n -doped semiconductors, respectively, used in conventional electronics [22] . The selectivity of these ion-conducting materials is a consequence of fixed ionic groups that are anchored to the polymer backbone of the material [15] . In a cation-selective material, such as an anionic polyelectrolyte, the anionic groups are fixed whereas the compensating cations are mobile. Mobile anions are repelled from entering the material by the high concentration of fixed anions (Donnan exclusion). An IBJT is formed by ionically connecting two channels of one type (labelled emitter (E) and collector (C)) with a channel of the other type (labelled base (B)) through a neutral polymer electrolyte ( Fig. 1 ). Two types of transistors can then be constructed, the npn -IBJT [14] ( Fig. 1a ) that conducts anions from the emitter to the collector, and the pnp -IBJT [4] ( Fig. 1b ) that instead conducts cations. Our transistors are fabricated on top of a polyethylene terephthalate substrate coated with the conductive polymer poly(3,4-ethylenedioxythiophene) poly(styrenesulfonate) (PEDOT:PSS) [23] . Through sequential photolithographic and etching steps, the structures are patterned and chemically modified to achieve the final device. The cation-selective layer is obtained by over-oxidizing [24] PEDOT:PSS, which terminates the electronic conductivity of the PEDOT phase while leaving the PSS phase intact. The anion selective layer consist of quaternized and crosslinked poly(vinylbenzylchloride) (PVBC) and the insulating layers are made from photopolymerized SU-8. Inkjetted poly(ethylene glycol) serves as the neutral polymer electrolyte and is capped by a drop of polydimethylsiloxane. The transduction from electronic to ionic signals occur at the PEDOT:PSS-Ag/AgCl electrodes covered with electrolyte ( Fig. 2a ). The Ag/AgCl paste partly covers the PEDOT:PSS and reduces the potential drop over the electrode from ~600 mV for a pure PEDOT:PSS electrode [14] to less than 25 mV ( Fig. 2b ). In the npn -IBJT anions diffuse through the polymer electrolyte junction (J) from the emitter to the collector. The rate of diffusion through the junction depends on the salt concentration within the junction, which is modulated by the base terminal. If cations are injected from the base, the salt concentration within the junction increases and the transistor junction is conductive. If the junction is depleted of cations by the base, it becomes nonconductive and only few anions can diffuse across it. The E, C and B channels exhibit ion resistances typically in the MΩ range that must be taken into account when designing circuits. Therefore, the sheet resistance of 50 and 200 μm wide n - and p -channels was measured ( Fig. 2c ). The desired resistance of each channel can then be obtained by choosing the length and width of the channel properly. 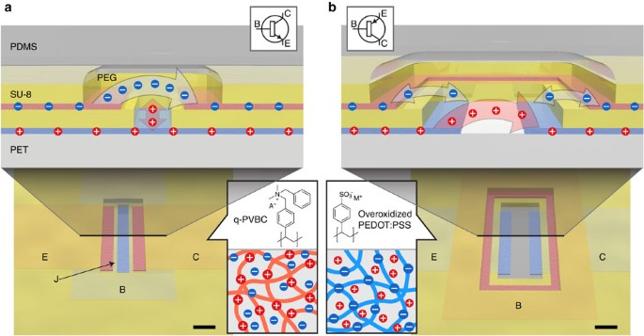Figure 1: Ion bipolar junction transistors. (a) In thenpn-IBJT anions come from the emitter (E), diffuses over the junction (J) and continue into the collector (C). The salt concentration within the junction, which governs the diffusion rate of anions, is modulated by the cationic current through the base (B). Emitter and collector consist of a crosslinked polycation and the base comprises a crosslinked polyanion. (b) In thepnp-IBJT, cations are transported between the emitter and collector whereas anions are transported through the base. Scale bars, 50 μm. Figure 1: Ion bipolar junction transistors. ( a ) In the npn -IBJT anions come from the emitter (E), diffuses over the junction (J) and continue into the collector (C). The salt concentration within the junction, which governs the diffusion rate of anions, is modulated by the cationic current through the base (B). Emitter and collector consist of a crosslinked polycation and the base comprises a crosslinked polyanion. ( b ) In the pnp -IBJT, cations are transported between the emitter and collector whereas anions are transported through the base. Scale bars, 50 μm. 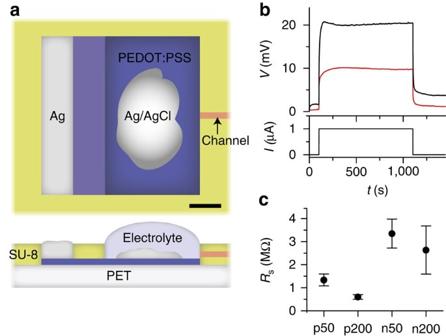Figure 2: Electrode configuration. (a) The redox active Ag/AgCl material is in electrical contact with the silver (Ag) connector through the PEDOT:PSS layer. An opening in the SU-8 layer confines the electrolyte and the electric current is converted into an ion current by redox reaction of the Ag/AgCl. The ion current goes into the chemical circuit through an ion conductive channel. The scale bar is 1 mm. (b) The voltage drop over the electrodes was measured in a three-electrode configuration. For the oxidized (black line) and reduced (red line) electrodes, the voltage drop was 20 mV and 10 mV, respectively. Most of the voltage drop disappeared within seconds after setting the current to zero. (c) The square resistance (RS) of 50 μm and 200 μm wide channels of both anion- (n) and cation (p)-selective type was measured. Mean values and standard deviations are presented withn=7. Full size image Figure 2: Electrode configuration. ( a ) The redox active Ag/AgCl material is in electrical contact with the silver (Ag) connector through the PEDOT:PSS layer. An opening in the SU-8 layer confines the electrolyte and the electric current is converted into an ion current by redox reaction of the Ag/AgCl. The ion current goes into the chemical circuit through an ion conductive channel. The scale bar is 1 mm. ( b ) The voltage drop over the electrodes was measured in a three-electrode configuration. For the oxidized (black line) and reduced (red line) electrodes, the voltage drop was 20 mV and 10 mV, respectively. Most of the voltage drop disappeared within seconds after setting the current to zero. ( c ) The square resistance ( R S ) of 50 μm and 200 μm wide channels of both anion- (n) and cation (p)-selective type was measured. Mean values and standard deviations are presented with n =7. Full size image Inverters Throughout the characterization of the ion logic gates, the supply voltage ( V CC ) was 10 V; thus, high input is defined as 10 V and low as 0 V. The output signal ( V O ) of an inverter (NOT gate) equals the inverted input signal ( V A ). Ideally, the output swing should be full, that is, V A =0 V gives V O =10 V and vice versa . In actual NOT gates, it is enough to have a forbidden voltage range separating high (logic 1) from low (logic 0); however, a large swing is still desirable. 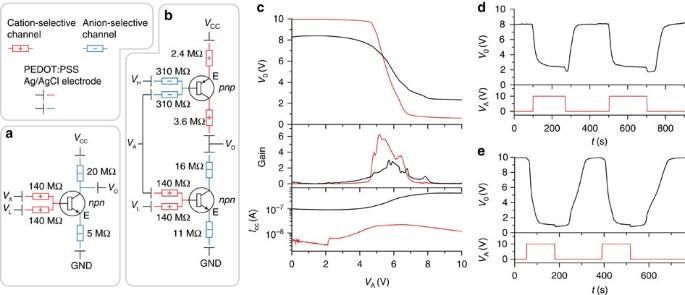Figure 3: Inverters based on IBJTs. (a) In thenpntype inverter, most of the supply voltage (VCC=10 V) is divided over thenpn-IBJT and the 20 MΩ resistance. For high input (VA=10 V), the transistor has low impedance and the output (VO) is high whereas the reverse happens for low input. (b) The complementary inverter is constructed by connecting anpn- and apnp-IBJT in series. (c) The swing and gain is better for the complementary inverter (red line) than for thenpntype inverter (black line). The supply current (ICC) is lower for the complementary inverter for which it reaches its maximum, during the switch between the end states. (d) The output voltage of thenpninverter for a pulse train as input. (e) The output voltage of the complementary inverter for a pulse train as input. Figure 3a shows the circuit diagram of an inverter based on a single npn -IBJT. The resistances in the circuit diagram were obtained from separate measurements on cation- and anion-selective channels ( Fig. 2c ). For a high input, the transistor has low impedance and most of the electric potential drop occurs over the top 20 MΩ ion resistor, thereby giving a low output signal. For a low input, the npn -IBJT is in its high impedance state and most of the potential drop occurs over it; thus, the output is high. As the impedance across the emitter-base junction is low in forward bias, the base resistance must be high. Unfortunately, the npn -IBJT requires a slightly negative base potential to be in its nonconductive state. This can be achieved by the addition of a pull-down voltage ( V L ) connected in parallel with the input terminal ( Fig. 3a ). For V L =−5 V, the base voltage is altered to the range of [−2.5, 2.5] V for [0, 10] V input signal (for I B =0 A). To improve the characteristics of the gate, the top 20 MΩ resistor may be replaced by a pnp -IBJT ( Fig. 3b ). In such complementary inverter, the npn -IBJT is nonconductive for a high input whereas the pnp -IBJT is nonconductive for a low-input signal. Together, this minimizes the power consumption of the NOT gate and improves its output swing (gain). To alter the base voltage of the pnp -IBJT, a pull-up voltage ( V H =15 V) has been added to the design. The input voltage was swept from 0 V to 10 V at a rate of 10 mV s −1 and the corresponding V O is shown in Fig. 3c . As expected, the output is initially high and starts to fall off towards the lower value at around 5 V. The high output of the npn inverter is ~8 V and is limited by the leakage current through the transistor in its nonconductive state. The low output reaches around 2.5 V and is limited by the potential drop over the 5 MΩ emitter resistor. For the complementary inverter, the high output reaches above 9.9 V and essentially the whole potential drop occurs over the nonconductive npn -IBJT as the pnp -IBJT is conductive. The low output reaches around 0.6 V and most of the potential drop occurs now instead across the nonconductive pnp -IBJT. In comparison, the swing is better for the complementary inverter than for the npn inverter, as expected. Also, the gain, which is defined as the absolute value of slope, is significantly higher for the complementary inverter. The gain must be above 1 to enable construction of functional logic circuits, and a higher gain is typically advantageous for a circuit′s performance. For the npn type inverter, the supply current ( I CC ) is low for low-input signals as the transistor is in its nonconductive state whereas I CC becomes higher for high input as the transistor is conductive in this state. For the complementary design, the ion current is low towards both the end states because one transistor is always nonconductive in these states, that is, at high or low V A values. The supply current reaches its maximum value during the switch when both transistors have relatively lower impedance. Figure 3d,e shows the switching transients for the npn and complementary inverters, respectively. The switching speed is slightly faster for the npn inverter whereas the swing is better for the complementary inverter. The inverters can be repeatedly switched in between the two states without any major change in output voltage levels. The delay time can be attributed to the migration of ions in and out from the neutral junction. It takes longer time to deplete the junction compared with injecting enough ions to make it conductive; thus, it takes longer to switch the npn inverter output signal from low to high than in the reverse direction. Figure 3: Inverters based on IBJTs. ( a ) In the npn type inverter, most of the supply voltage ( V CC =10 V) is divided over the npn -IBJT and the 20 MΩ resistance. For high input ( V A =10 V), the transistor has low impedance and the output ( V O ) is high whereas the reverse happens for low input. ( b ) The complementary inverter is constructed by connecting a npn - and a pnp -IBJT in series. ( c ) The swing and gain is better for the complementary inverter (red line) than for the npn type inverter (black line). The supply current ( I CC ) is lower for the complementary inverter for which it reaches its maximum, during the switch between the end states. ( d ) The output voltage of the npn inverter for a pulse train as input. ( e ) The output voltage of the complementary inverter for a pulse train as input. Full size image NAND gates The designs of npn -IBJT type NAND and complementary NAND gates are shown in Fig. 4a,b , respectively. The difference between the two designs is that the high resistor in the npn type design has been replaced by two pnp -IBJTs connected in parallel in the complementary design. In theory, this should allow for better swing as the pnp -IBJTs can change their impedance. To evaluate the NAND gates, the two input signals V A and V B were switched between high and low to probe all four possible states ( Fig. 4c ). The npn type NAND has high and low output levels of 6 and 2 V, respectively. The lower level is quite close to the limit imposed by the voltage division across the resistors in the circuit. The upper limit, however, is limited by the state in which one of the transistors is conductive while the other one is nonconductive. A possible explanation for this is that one conductive transistor decreases the combined impedance and that the base current of this conductive transistor contributes to the voltage drop. The complementary NAND gate does not suffer such a pronounced voltage drop, when one of the input signals is high ( Fig. 4d ). For this gate, the high-and-low output levels are 7.5 V and 3.5 V, respectively. Here the upper level is relatively good whereas the lower level is unfortunately rather high. This might be attributed to sub-optimal function of the pnp -IBJTs as the leakage current becomes worse when they are connected in parallel. 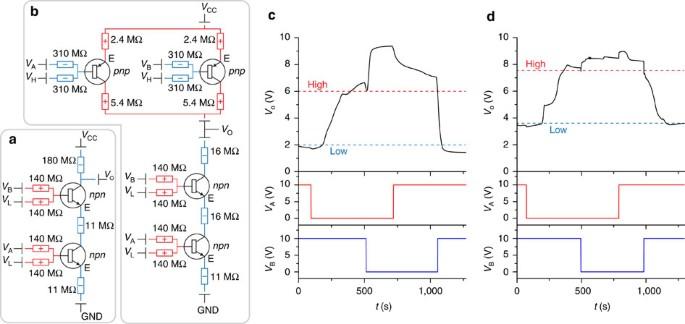Figure 4: NAND gates based on IBJTs. (a) Thenpntype NAND gate (NAND) comprises twonpn-IBJTs and one large resistor connected in series. (b) In the complementary NAND gate (CNAND), the large resistor has been replaced by twopnp-IBJTs connected in parallel. (c) The response of the NAND gate to the four possible combinations of input (VA,VB). The high-and-low output levels for the supplied input signals are marked with dashed lines. (d) The response of the CNAND gate to the four possible combinations of input. Figure 4: NAND gates based on IBJTs. ( a ) The npn type NAND gate (NAND) comprises two npn -IBJTs and one large resistor connected in series. ( b ) In the complementary NAND gate (CNAND), the large resistor has been replaced by two pnp -IBJTs connected in parallel. ( c ) The response of the NAND gate to the four possible combinations of input ( V A , V B ). The high-and-low output levels for the supplied input signals are marked with dashed lines. ( d ) The response of the CNAND gate to the four possible combinations of input. Full size image In this work, we have demonstrated for the first time, to our knowledge, npn type and complementary logic gates based on ion transistors. The integration of several transistors onto one chip is an important step towards future applications for chemical circuits, as the vast majority of those require multiple transistor configurations. The fabrication of the previously reported pnp -IBJTs included a manual lamination step, which has been eliminated by a new design with photolithographic patterning of the anion-selective channels, which makes the fabrication of pnp -IBJTs identical to that of npn -IBJTs. Thus, the fabrication process employed here allows for manufacturing of more complex integrated ion circuits without any major modifications. The reported inverters and NAND gates exhibit a gain and operational voltage window characteristics that promise for the construction of integrated circuits. One concern with the present ion logic circuits, however, is the rather low switching speed. The time required to fully switch the inverters is in the order of 100 s and it depends primarily on the amount of injected/extracted charge ( Q ) that needs to pass through the base. The concentration profile within the junction can be approximated by a linear gradient [4] with concentration c E at the emitter and zero concentration at the collector. The collector current I C c E /L ( L is the emitter-collector spacing); thus, the required Q for a specific I C and L is Q c E L I C L. [2] So, by reducing the present emitter-collector spacing from 50 to 5 μm would thus render the switching time to decrease down to 1 s. Therefore, we believe that a reduction of the circuit dimensions, that is, line widths and channel lengths, would render switching times below 1 s possible. Miniaturization of the current system faces challenges, mainly arising from the shrinking of the flexible substrate during processing, which introduces alignment errors. Another feasible route to improve the switching speed would be to increase the ion mobility within the junction. Again assume a linear concentration gradient between the emitter and the collector [4] , with the concentration c E above and at the edge of the emitter. As the concentration is close to zero at the collector, the limiting current density [15] through the junction can be written as j L =2RTμ − c E /L where R is the gas constant, T is the temperature, μ − is the mobility of the anionic species and L is the emitter-collector spacing. The amount of salt within the junction can be obtained by integrating the extraction current throughout the base when switching the IBJT from active mode to cutoff mode. The extracted amount of charge Q relates to the concentration at the emitter by Q =( c E L E +c E L/2)AF where L E is the length of the emitter within the junction, F is the Faraday constant and A is the cross-section area of the junction. Thus, μ − = j L L/(2RTQ/(AF(L E +L/2))) = j L ALF(L E +L/2)/(2RTQ) = I C LF(L E +L/2)/(2RTQ) . For the previously published npn -IBJT [14] Q =1.8 μC for I C =244 nA, which gives μ Cl− =2×10 −4 cm 2 Vs −1 , a value only 4 times lower than the mobility in water. Thus, no major improvement of the mobility is possible as the junction is well hydrated. In biological, chemical and medical applications, there is a need for a technology to gate and distribute chemical signals and to alter gradients along for instance the floor of a Petri dish or a cell growth plate. Our findings promise for areal 2D cross-point circuits in which addressing and release of chemicals can be achieved via X–Y addressing. As the development continues of chemical circuits, we envisage future applicability of this technology to fields which deals with transport of ions and biomolecules [25] , [26] , [27] , [28] . Manufacturing Detailed device structures are shown in Supplementary Fig. S1 . A plastic polyethylene terephthalate foil coated with a thin layer of poly(3,4-ethylenedioxythiophene):poly(styrenesulfonate) (PEDOT:PSS) was used as substrate (AGFA-Gevaert Orgacon F-350). To promote adhesion, the substrate was cleaned with Shipley 1112A remover, rinsed in acetone and deionized water, baked (110 °C, 10 min), reactive-ion etched in O 2 -plasma (150 W, 8 s) and coated with primer (hexamethyldisilazane). Shipley s1805 photoresist was spin-coated onto the substrate that sequentially was exposed with a mask aligner (Suss MA/BA 6) and developed in Microposit MF319. After baking (110 °C, 10 min), the pattern was dry-etched with O 2 /CF 4 plasma (reactive-ion etched, 150 W, 20 s) and the remaining photoresist was removed (Shipley 1112A). Another photoresist layer was patterned (Shipley s1813) where the openings were overoxidized (aqueous sodium hypochlorite solution, 1% (vol/vol), 120 s). The substrate was cleaned with remover, rinsed and baked (110 °C, 20 min). Next, a layer of SU-8 2010 (MicroChem) was patterned according to manufacturer′s instructions. A new Shipley s1818 photoresist layer was patterned to protect the PEDOT:PSS electrodes. After baking (110 °C, 30 min), the anion exchange membrane solution (see below) was spin-coated (1500 r.p.m.) and baked (110 °C, 45 min). A protective poly(methyl methacrylate) (30 mg ml −1 ) layer was spin-coated (3,000 r.p.m.) before a photoresist layer was patterned and etched (O 2 /CF 4 plasma, 100 s). After photoresist removal and rinsing, a SU-8 2010 encapsulation layer with openings for the electrodes and junctions was patterned. Poly(ethylene glycol) (mol wt 950–1,050, 500 mg ml −1 in cyclopentanone) was printed into the junctions with a Dimatix inkjet printer (DMP-2800). The junctions were sealed with drops of polydimethylsiloxane (10:1 Sylgard 186, cured at 100 °C for 1 h). Silver contacts and silver/silver chloride (Ag/AgCl, Advanced materials 500) electrodes were painted on top of the PEDOT:PSS electrodes and cured at 110 °C for 15 min. Anion exchange membrane solution The reaction scheme utilized in this work was a modified version of the one reported by Pandey et al . [29] PVBC (60/40 mixture of 3- and 4-isomers, Mn ~55,000 and Mw ~100,000) and diazabicyclo[2.2.2]octane (DABCO, >99%) were purchased from Sigma-Aldrich and N-benzyldimethylamine (>98%) was purchased from Alfa Aesar. A mixture of PVBC (500 μl, 200 mg ml −1 dissolved in tetrahydrofuran) and N -benzyldimethylamine (76 μl) was heated in a water bath (50 °C, 1 h). The precipitate was rinsed in acetone and thereafter dissolved in 1 ml deionized water. Immediately before use, 1-propanol (1 ml) and DABCO (6.6 μl, 5 M in ethanol) was added to the mixture. Electrical characterization The devices were soaked in deionized water for at least 24 h before use. Aqueous 0.1 M NaCl solution was used as electrolyte and presented data was obtained after stable operation had been reached (typically after five switches). Electrical measurements were recorded with one Keithley 2602A and two Keithley 2400 source meters controlled via LabVIEW (sample rate 1 Hz). In addition, two simple power supplies were used for the pull up/down voltages. Adjacent-averaging was used on characterization data to reduce noise. How to cite this article: Tybrandt, K. et al . Logic gates based on ion transistors. Nat. Commun. 3:871 doi: 10.1038/ncomms1869 (2012).